Deglacial water-table decline in Southern
                            California recorded by noble gas isotopes 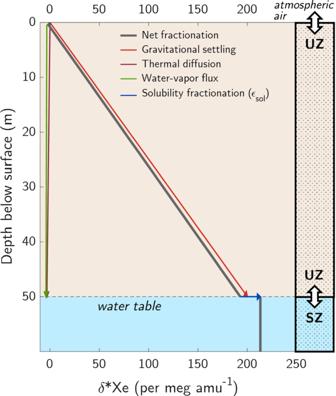Fig. 1: Steady-state xenon isotopic fractionation
                                                  in an unconfined aquifer. Gravitational settling causes mass
                                                  difference-normalized, heavy-to-light xenon
                                                  isotope ratios (δ*Xe) in unsaturated zone (UZ) air
                                                  to increase with depth below the land surface,
                                                  relative to atmospheric air. At the water table,
                                                  dissolved gases in the saturated zone (SZ)
                                                  equilibrate with deep UZ air. Solubility
                                                  fractionation causes δ*Xe to further increase in
                                                  the dissolved phase relative to the gas phase.
                                                  Note that nearly all water-vapor flux
                                                  fractionation occurs between the surface and
                                                  shallow wetting front (at one meter depth in this
                                                  idealized illustration), below which water-vapor
                                                  flux fractionation is nearly constant with depth
                                                  and only changes due to its weak sensitivity to
                                                  temperature12,13. Constraining the magnitude of past hydrological change
                                may improve understanding and predictions of future shifts in water
                                availability. Here we demonstrate that water-table depth, a
                                sensitive indicator of hydroclimate, can be quantitatively
                                reconstructed using Kr and Xe isotopes in groundwater. We present
                                the first-ever measurements of these dissolved noble gas isotopes in
                                groundwater at high precision (≤0.005‰
                                    amu −1 ; 1σ), which reveal
                                depth-proportional signals set by gravitational settling in soil air
                                at the time of recharge. Analyses of California groundwater
                                successfully reproduce modern groundwater levels and indicate a
                                17.9 ± 1.3 m (±1 SE) decline in water-table depth in Southern
                                California during the last deglaciation. This hydroclimatic
                                transition from the wetter glacial period to more arid Holocene
                                accompanies a surface warming of 6.2 ± 0.6 °C (±1 SE). This new
                                hydroclimate proxy builds upon an existing paleo-temperature
                                application of noble gases and may identify regions prone to future
                                hydrological change. Noble gases dissolved in groundwater have a wide range
                                of physical applications for climatology and hydrogeology, owing to
                                their chemical and biological inertness. For example, past
                                mean-annual surface temperatures derived from noble gases in
                                paleo-groundwater comprise some of the most reliable terrestrial
                                temperature reconstructions of the last glacial
                                        period [1] , [2] . Physical models of
                                groundwater recharge, transport, contamination, and age also are
                                frequently constrained by noble gas
                                        measurements [3] , [4] , [5] . Although dissolved noble gas
                                concentrations and helium isotopes are routinely measured,
                                groundwater Kr and Xe stable isotope studies are rare because
                                fractionation signals are generally smaller than typical order 1–10‰
                                    amu −1 analytical
                                uncertainties. Here we apply a newly developed
                                        technique [6] to make the first-ever
                                measurements of stable Kr and Xe isotope ratios in groundwater at
                                high precision (≤5 per meg amu −1 /1σ;
                                where 1 per meg = 0.001‰ = 0.0001%). Measurement of Kr and Xe
                                isotope ratios, along with Ar isotopes and Ar, Kr, and Xe
                                concentrations, in 58 groundwater samples from 36 wells allowed us
                                to test a simple fractionation model constrained by recent
                                experimental determinations of noble gas isotopic solubility and
                                diffusivity ratios [6] . Our findings suggest that Kr
                                and Xe isotope ratios in groundwater record the depth to water at
                                the time and place of recharge. We present an inverse model to
                                reconstruct past water-table depth (WTD) based on noble gas
                                measurements and demonstrate its accuracy in reproducing observed
                                water levels in modern groundwater. We then apply it to a suite of
                                paleo-groundwater samples from San Diego, California, which indicate
                                a ~20-m decline in reconstructed WTD during the last deglaciation. We interpret this shift as a regional groundwater response to a
                                major hydroclimatic change from the wetter glacial period to more
                                arid Holocene. This finding is consistent with previous
                                paleo-hydrological evidence and climate model simulations from the
                                southwestern United States [7] , [8] , [9] , [10] , [11] . Depth-dependent gravitational isotopic signals A theoretical model for gas-phase isotopic
                                    fractionation in porous media, validated by soil air
                                    observations, suggests that dissolved Kr and Xe stable isotope
                                    ratios in unsaturated-zone (UZ) air are primarily fractionated
                                    from the well-mixed atmosphere by gravitational
                                            settling [12] , [13] . Gravitational settling
                                    is a well understood process by which molecular diffusion in
                                    stagnant air in hydrostatic balance leads to a nearly linear
                                    increase in heavy-to-light gas ratios with
                                            depth [14] . Past measurements of
                                    inert gases in polar firn [15] , [16] and UZ
                                            air [12] , [13] have been found to be in
                                    close agreement with the theoretical gravitational settling
                                    slope (e.g. ~4.0 per meg
                                        amu −1 m −1 at ~20 °C). Thermal diffusion [17] and
                                    steady-state UZ-to-atmosphere water-vapor
                                            fluxes [12] both weakly oppose the
                                    influence of gravitational settling on UZ air isotopic
                                    composition (Fig. 1 ). In
                                    the presence of a temperature gradient, thermal diffusion acts
                                    to concentrate heavy gases towards the cooler end of a column of
                                    gas. Thermal diffusion decreases heavy-to-light isotope ratios
                                    in deep UZ air, which is warmed by geothermal heat from below,
                                    relative to the atmosphere. Isotope ratios of the lighter noble
                                    gases (He, Ne, and Ar) are more strongly affected by thermal
                                    diffusion than Kr and Xe isotope ratios, per mass unit
                                            difference [18] , [19] . At steady-state, the
                                    flux of water vapor from the moist UZ to drier overlying surface
                                    air leads to a kinetic isotopic fractionation that also lowers
                                    heavy-to-light isotope ratios and affects the lighter noble
                                    gases more than Kr and Xe [12] , [13] . This
                                    fractionation is induced by vertical partial pressure gradients
                                    of dry air constituents between the atmosphere and UZ, which
                                    drive steady-state molecular diffusion of atmospheric noble
                                    gases into the UZ against the upwards flux of water
                                            vapor [12] . Fig. 1: Steady-state xenon isotopic fractionation
                                                  in an unconfined aquifer. Gravitational settling causes mass
                                                  difference-normalized, heavy-to-light xenon
                                                  isotope ratios (δ*Xe) in unsaturated zone (UZ) air
                                                  to increase with depth below the land surface,
                                                  relative to atmospheric air. At the water table,
                                                  dissolved gases in the saturated zone (SZ)
                                                  equilibrate with deep UZ air. Solubility
                                                  fractionation causes δ*Xe to further increase in
                                                  the dissolved phase relative to the gas phase. Note that nearly all water-vapor flux
                                                  fractionation occurs between the surface and
                                                  shallow wetting front (at one meter depth in this
                                                  idealized illustration), below which water-vapor
                                                  flux fractionation is nearly constant with depth
                                                  and only changes due to its weak sensitivity to
                                                  temperature [12] , [13] . Full size image Air at the bottom of the UZ dissolves into
                                    groundwater at the water table, thereby transferring the signal
                                    of UZ air fractionation to dissolved isotope ratios in
                                    groundwater, as depicted in an idealized model of an unconfined
                                    aquifer system (Fig. 1 ). Small isotopic solubility differences, constrained by recent
                                            determinations [6] , lead to slight further
                                    increases of heavy-to-light isotope ratios. Over time, as the
                                    uppermost groundwater is gradually displaced downward by
                                    subsequent recharge, it is sequestered from overlying UZ air,
                                    prohibiting further gas exchange. After the time of recharge,
                                    which is here defined to be the last period of contact between a
                                    groundwater parcel and overlying UZ air, the dissolved noble gas
                                    composition is retained except for dispersive intra-aquifer
                                    mixing. Therefore, the noble gas composition of old groundwater
                                    reflects conditions set at the water table at the time and place
                                    of recharge [20] , [21] . In this conceptual framework, a dissolved isotope
                                    ratio ( δ diss ) is cumulatively
                                    fractionated at the time of recharge from its atmospheric ratio
                                        ( δ atm , where δ atm = 0 by
                                    definition) by steady-state diffusive processes in UZ air
                                        ( ε UZ ), isotopic solubility
                                    fractionation ( ε sol ), and the injection
                                    of excess air arising from the dissolution of entrapped soil air
                                    bubbles ( ε EA ): 
    δ _diss = ε _UZ + ε _sol + ε _EA
 (1) Solubility fractionation refers to the preferential
                                    dissolution of heavy Kr and Xe isotopes, versus light isotopes,
                                    in fresh water at solubility
                                            equilibrium [6] . The isotopic influence
                                    of excess air opposes that of solubility fractionation by an
                                    amount that depends on the quantity of initially entrapped soil
                                    air and the completeness of its dissolution under the assumption
                                    of a closed water-bubble system at solubility
                                            equilibrium [2] . A recent study of
                                    solubility and kinetic fractionation of Kr and Xe isotopes in
                                    fresh water demonstrated that ε EA is negligible (order
                                    1 per meg amu −1 ) and ε sol is
                                    largely insensitive to temperature [6] . In
                                    principle, therefore, differences between dissolved Kr and Xe
                                    isotope ratios in groundwater and atmospheric air should
                                    primarily arise from only two processes: gravitational settling,
                                    which is the primary control on ε UZ , and solubility
                                    fractionation (Fig. 1 ). High-precision Kr and Xe isotope measurements in
                                    groundwater To test this expectation, we compare the mass
                                    difference-normalized, error-weighted means of Kr and Xe
                                    heavy-to-light isotope ratios (δ*Kr and δ*Xe, respectively) in
                                    58 groundwater samples collected from three regions in
                                    California: Fresno, the Mojave Desert, and San Diego
                                        (Fig. 2 ). Because
                                    gravitational settling depends only on isotopic mass difference,
                                    it leads to an identical increase in these mass
                                    difference-normalized isotope ratios with depth (i.e. δ*Kr and
                                    δ*Xe will covary with a slope of 1 if fractionated only by
                                    gravitational settling). Fig. 2: Dissolved Kr and Xe isotope ratios in
                                                  groundwater. Isotope ratio measurements in 58
                                                  groundwater samples collected from 36 wells
                                                  illustrate the dominance of gravitational settling
                                                  in driving isotopic departures from solubility
                                                  equilibrium. Mojave Desert samples for which δ*Kr
                                                  exceeds 200 per meg
                                                  amu −1 are shown both as
                                                  original values (open circles) and corrected for
                                                  fractionation due to oxygen consumption
                                                  (Supplemental Note 5 ). Error bars indicate ±2-σ
                                                  uncertainty. Inset: predicted fractionation
                                                  associated with (1) two meters of gravitational
                                                  settling; (2) thermal diffusion caused by a 2 °C
                                                  difference between the surface and water table
                                                  (WT); (3) a steady-state WT-to-atmosphere
                                                  water-vapor flux driven by a 0.81% WT-atmosphere
                                                  absolute humidity difference (equivalent to 20 °C,
                                                  65% relative humidity surface air); (4) complete
                                                  dissolution of entrapped soil air bubbles
                                                  (equivalent to 50% ΔNe); and (5) steady-state
                                                  oxygen depletion leading to a 0.5%
                                                  atmosphere-to-deep unsaturated zone difference in
                                                  the sum of O 2 and
                                                  CO 2 . Note that the inset
                                                  scale is magnified. Full size image Indeed, we find that δ*Kr and δ*Xe in all samples
                                    are greater than or equal to ε sol , and a linear
                                    regression through all measurements has a slope of 1.16 ± 0.02
                                        ( R 2 = 0.98). The 40
                                    Fresno and San Diego samples fall along a linear trendline with
                                    a slope of 1.03 ± 0.04 that originates at the solubility
                                    equilibrium value. As described above, other non-gravitational
                                    isotopic fractionation processes in UZ air and groundwater
                                    generally exhibit different δ*Kr vs. δ*Xe slopes from
                                    gravitational settling and are both opposite in sign and smaller
                                    in magnitude. For context, as little as two meters equivalent of
                                    gravitational settling fractionation in UZ air exceeds the
                                    expected individual magnitudes of Kr and Xe isotopic
                                    fractionation associated with each of the following: thermal
                                    diffusion driven by a 2 °C water-table-to-surface temperature
                                    difference, a steady-state water-vapor flux from the moist UZ
                                    into 20 °C, 65% relative humidity surface air, and complete
                                    dissolution of entrapped soil air bubbles yielding excess air
                                    equivalent to 50% Ne supersaturation (ΔNe; Fig. 2 ). Mojave Desert groundwater samples exhibit slight
                                    departures from the expected concordant Kr and Xe relationship
                                    that are most apparent in samples collected from regions of deep
                                    present-day water table depths (>50 m). We suspect that an
                                    additional physical process systematically affects these deep
                                    samples. Two candidate mechanisms are disequilibrium kinetic
                                            fractionation [18] driven by barometric
                                    pumping or oxygen consumption [22] , [23] without
                                    equimolar replacement by CO 2 in deep UZ
                                    air (Supplementary Note 5 ). We explored a simple model for the latter
                                    process, in which the mole fractions of
                                        O 2 and CO 2 in
                                    deep UZ air above the water table together comprise ~16% of dry
                                    air. This is equivalent to a 5% depletion from the overlying
                                    atmosphere, in which O 2 and
                                        CO 2 comprise ~21% of dry air. This 5%
                                    depletion falls within the observed range of
                                        O 2 consumption in past UZ air
                                            studies [22] , [23] and may explain the
                                    discordant Mojave Desert data, as illustrated in
                                        Fig. 2 . Inferring WTD from dissolved δ*Kr and δ*Xe The close agreement of groundwater δ*Kr and δ*Xe
                                    with the expected gravitational slope is encouraging for
                                    quantitative reconstruction of past WTD based on isotopic
                                    measurements. To explore this possible application, we developed
                                    an inverse model that estimates past WTD, recharge temperature,
                                    and excess air parameters [2] constrained by measured noble gas isotope ratios and elemental
                                    concentrations. With knowledge of both recharge temperature and
                                    WTD, it is now possible to quantify and remove the contributions
                                    of UZ fractionation and geothermal heat to reconstructions of
                                    past surface temperature, thereby resolving two longstanding
                                    concerns about noble gas
                                            paleo-thermometry [20] . Our
                                    inverse model approach merges existing models for equilibrium
                                    dissolution and excess air [2] and UZ
                                    air fractionation [13] in an iterative loop
                                    that converges on best estimates of WTD and temperature
                                    (Supplementary Fig. 2 ). Analytical measurement uncertainties are
                                    propagated to estimate probability distributions of WTD and
                                    temperature via Monte Carlo simulations. We first tested this inverse model with five
                                    samples collected from two Fresno wells of relatively young
                                    recharge age, ~650 and ~35 years, which were constrained by
                                    multiple independent dating tools
                                        ( 3 H/ 3 He,
                                        SF 6 , and 85 Kr, 14 C, and 39 Ar). Using measured Ar, Kr, and
                                    Xe isotope ratios and elemental concentrations, we reconstructed
                                    WTDs for comparison with nearby historical water-level
                                    observations. The younger samples, which have a mean recharge
                                    year of 1983 CE (±5 years), agree closely with the mean of
                                    nearby water-level observations in the early 1980s
                                        (Fig. 3 ). The older
                                    samples fall within the range of decadal variability prior to
                                    1950, before major development of the Fresno region, and likely
                                    reflect mean mid-to-late Holocene regional WTD due to smoothing
                                    of isotopic signals by dispersive mixing (Supplementary
                                        Note 3 ). Fig. 3: Modern validation of noble gas
                                                  isotope-derived water table depths. Water-table depth estimates derived from
                                                  groundwater noble gas isotope measurements are
                                                  compared to historical water-level observations
                                                  near two adjacent wells sampled in March 2018 near
                                                  Fresno, California. Depths are relative to the
                                                  land surface. Historical records from within a
                                                  10-km radius of the sample site were included,
                                                  except for those from the highly populated city
                                                  center, which dropped substantially in the
                                                  mid-20th century (Supplementary Fig. 4 ). Multiple age
                                                  tracers were used to determine probable recharge
                                                  ages (Supplementary Fig. 5 ). Full size image Reconstructing past hydroclimatic shifts in WTD To investigate the potential for WTD reconstruction
                                    as a novel tool for paleoclimate, we collected and analyzed
                                    samples from 23 San Diego monitoring wells, 18 of which contain
                                    groundwater from a confined regional aquifer system with 14 C-dated recharge ages between
                                    5 ka and 40 ka (Supplementary Note 4 ). Here we consider noble gas isotopes and
                                    concentrations in samples collected from these 18 monitoring
                                    wells, which individually provide access to groundwater at
                                    various depths at six separate locations in the western portion
                                    of the recharge area (Fig. 4 inset). The regional groundwater system
                                    flows from east to west and is presumed to recharge over
                                    high-permeability alluvial deposits near stream channels west of
                                    the mountainous topography and crystalline surficial geology
                                    that characterize the region 10–15 km east of the well sites
                                    (Supplementary Note 4 ). Fundamentally, paleoclimate reconstruction
                                    using groundwater relies on an understanding that dispersive
                                    intra-aquifer mixing of groundwater originating from various
                                    times and places of recharge smooths climatic signals and acts
                                    as an effective spatiotemporal low-pass
                                            filter [20] . Therefore, we primarily
                                    expect low-frequency climatic signals to be preserved by noble
                                    gases in groundwater, which thus provide high quality
                                    information about long-term changes in mean regional WTD and
                                    temperature across a major climate transition such as the last
                                        deglaciation. Fig. 4: Reconstructed water-table depths in the San
                                                  Diego region. Noble gas isotope-derived water-table
                                                  depths (WTD) from the San Diego aquifer system are
                                                  presented in meters below the land surface. Blue
                                                  markers and error bars (±2σ) indicate WTD derived
                                                  from individual samples collected from wells at
                                                  multiple depths at six sites (indicated by marker
                                                  shapes). Pre and post 15-ka mean WTDs (lines with
                                                  ±2-SE shaded regions) exclude two extreme WTD
                                                  observations that could reflect a previously
                                                  documented glacial dry period and wet Younger
                                                  Dryas stadial. The present-day mean WTD over the
                                                  assumed recharge area (inset) was estimated by a
                                                  high-resolution, observation-constrained
                                                  groundwater model (red square marker). Groundwater
                                                  age uncertainties are roughly ±2 ka (Supplementary
                                                  Note 4 ). Full size image As shown in Fig. 4 , Kr and Xe isotope-based reconstructions
                                    reveal considerably shallower WTDs throughout the latter portion
                                    of last glacial period (LLGP; defined here as 15–40 ka) before
                                    deepening during the last deglaciation (Fig. 4 ). Excluding samples from two
                                    outlier wells discussed below, we find mean regional WTDs during
                                    the LLGP and post-LLGP of 21.1 ± 0.8 m (±1 SE; 20 samples from
                                    11 wells) and 39.1 ± 1.0 m (±1 SE; 6 samples from 5 wells),
                                    respectively, indicating a deglacial WTD decline of 17.9 ± 1.3 m
                                    (±1 SE). Our finding of a shallower mean WTD during the LLGP is
                                    consistent with previous paleoclimate proxy reconstructions and
                                    model simulations [7] , [8] , [9] , [10] , [11] , which have suggested
                                    that glacial-period wintertime storm tracks were displaced
                                    southward due to interaction of the mean atmospheric circulation
                                    over western North America with the Laurentide Ice Sheet (LIS),
                                    delivering enhanced rainfall to the southwestern United States. A decline in WTD during the last glacial termination is
                                    indicative of a shift towards drier conditions, possibly linked
                                    to a northward migration of the wintertime storm tracks in
                                    response to the receding LIS. Although smoothing of abrupt
                                    climate signals in groundwater by dispersive
                                            mixing [20] precludes placing tight
                                    constraints on the timing of the deglacial WTD shift, the
                                    apparent timing of roughly 15 ka is temporally consistent with
                                    the rapid lowering of the LIS [24] . Simulation of mean WTD over an assumed recharge area by a
                                    high-resolution groundwater model [25] indicates a present-day regional-mean WTD of 47 m, which is
                                    substantially below the 21 m LLGP-mean WTD. Although topographic
                                    variability leads to spatial inhomogeneity in WTD, we suggest
                                    that dispersive mixing integrates isotopic WTD signals from
                                    water recharged over a wide spatial range and may therefore damp
                                    variability arising from spatial differences in topography. The
                                    close agreement of samples from 11 of 12 total LLGP wells
                                    supports the notion that the observed change in WTD reflects a
                                    regionally coherent groundwater response to a major
                                    hydroclimatic shift. 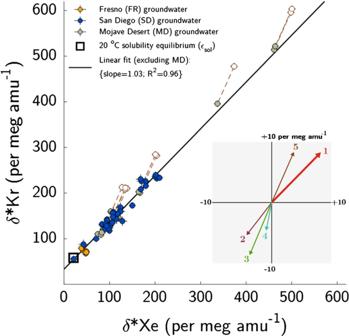Fig. 2: Dissolved Kr and Xe isotope ratios in
                                                  groundwater. Isotope ratio measurements in 58
                                                  groundwater samples collected from 36 wells
                                                  illustrate the dominance of gravitational settling
                                                  in driving isotopic departures from solubility
                                                  equilibrium. Mojave Desert samples for which δ*Kr
                                                  exceeds 200 per meg
                                                  amu−1are shown both as
                                                  original values (open circles) and corrected for
                                                  fractionation due to oxygen consumption
                                                  (Supplemental Note5). Error bars indicate ±2-σ
                                                  uncertainty. Inset: predicted fractionation
                                                  associated with (1) two meters of gravitational
                                                  settling; (2) thermal diffusion caused by a 2 °C
                                                  difference between the surface and water table
                                                  (WT); (3) a steady-state WT-to-atmosphere
                                                  water-vapor flux driven by a 0.81% WT-atmosphere
                                                  absolute humidity difference (equivalent to 20 °C,
                                                  65% relative humidity surface air); (4) complete
                                                  dissolution of entrapped soil air bubbles
                                                  (equivalent to 50% ΔNe); and (5) steady-state
                                                  oxygen depletion leading to a 0.5%
                                                  atmosphere-to-deep unsaturated zone difference in
                                                  the sum of O2and
                                                  CO2. Note that the inset
                                                  scale is magnified. For the first time, we are able to reconstruct
                                    surface temperature by accounting for both geothermal heat and
                                    UZ air fractionation in the San Diego regional aquifer samples. We find that the mean temperature during the LLGP was
                                    13.6 ± 0.2 °C (±1 SE) before warming to 19.9 ± 0.5 °C (±1 SE) in
                                    the Holocene, which closely matches modern regional surface
                                    temperatures (Supplementary Fig. 8 ). Two San Diego multiple-depth well sites
                                    exhibit high apparent LLGP recharge temperatures, which may have
                                    a geothermal origin or may indicate adsorption (Supplementary
                                        Fig. 9 ) and are
                                    thus excluded from our surface temperature analysis. We
                                    demonstrate that any effect on Kr and Xe isotopes in these two
                                    samples, and therefore on WTD estimation, is negligible
                                    (Supplementary Note 4 ,
                                    Supplementary Fig. 10 ). Two wells with outlier reconstructed WTDs have
                                    apparent 14 C-based recharge ages of
                                    ~24 ka and 12 ka, which may be temporally consistent with other
                                    studies that have proposed evidence for a local glacial
                                    megadrought and wet Younger Dryas stadial, respectively. Measurements of various physical, geochemical, and biological
                                    proxies from Lake Elsinore, roughly 100 km north of our SD study
                                    area, independently suggest extreme aridity persisting from
                                    ~27.5 to 25.5 ka [26] , [27] , [28] , which is within the
                                    dating uncertainty of the ~24 ka groundwater sample. A record of
                                    groundwater-discharge deposits from southeastern Arizona
                                    suggests the persistence of a shallow, near-surface regional
                                    water table from ~50 ka to 15 ka, after which the water-table
                                    lowered, except for a brief rebound to wet conditions during the
                                    Younger Dryas stadial ~12.5 ka [29] . Although reconstructed WTDs from these San Diego wells in
                                    principle support the notions of regional dry and wet periods
                                    around 24 ka and 12 ka, respectively, we cannot be certain that
                                    these reconstructed WTDs represent climatic signals rather than
                                    anomalous hydrogeological conditions. Similarly, the
                                    preservation of climatic signals from these periods would
                                    require minimal dispersive mixing along the flow path, which we
                                    cannot conclude based on our limited knowledge of the
                                    groundwater flow system. Future outlook on water-table depth
                                    reconstruction Based on the observed concordance of Kr and Xe
                                    isotopic measurements in groundwater with the expected primary
                                    influence of depth-dependent gravitational signals, we suggest
                                    that these measurements represent a promising new tool for
                                    hydrogeology and paleoclimatology. By analyzing dissolved Kr and
                                    Xe isotope ratios at high precision for the first time, we have
                                    (a) confirmed the dominant role of UZ gravitational settling in
                                    setting dissolved Kr and Xe isotope ratios in groundwater, (b)
                                    found close agreement between observed and reconstructed WTDs in
                                    Fresno samples of recent recharge, and (c) quantified a
                                    pronounced decrease in San Diego regional WTD during the last
                                    deglaciation. While future experiments may shed light on small
                                    departures from gravitational expectation as seen in the Mojave
                                    Desert samples, our findings offer strong support for the notion
                                    that heavy noble gas isotopes in groundwater are quantitative
                                    recorders of WTD at the time of recharge. Knowledge of past WTD
                                    not only provides an important correction to groundwater noble
                                    gas paleo-temperature reconstruction, but also adds
                                    complementary hydroclimate information. Future applications to
                                    constrain regional-scale groundwater flow models may enable
                                    quantitative reconstruction of past
                                    precipitation-minus-evaporation rates and improve our
                                    understanding of groundwater hydrogeology in aquifer systems
                                    presently supporting large populations. Groundwater sampling In this study, a total of 58 groundwater samples
                                    from 36 wells were collected in evacuated two-liter flasks and
                                    analyzed in the Scripps Institution of Oceanography (SIO) Noble
                                    Gas Isotope Laboratory. The borosilicate glass flasks used in
                                    this study were made to include two necks leading to 9-mm
                                    diameter Louwers-Hapert valves with double o-ring inner and
                                    outer seals. Sampling flasks were prepared, stored, and filled
                                    following procedures described in Seltzer et
                                            al. [6] , which are based on
                                    seawater dissolved gas sampling
                                            techniques [30] . Before and after sample
                                    collection, the necks and cavities between the inner two o-rings
                                    were flushed with nitrogen gas before the cavities were sealed
                                    and necks closed off with rubber caps. All samples were
                                    collected within 5 days of evacuation and analyzed within 2
                                    weeks of collection. A comparison of replicate sample
                                    differences in
                                        δ 40 / 36 Ar
                                    across 1 year of distilled water, groundwater, and seawater
                                    sample analyses, including those in this study, revealed no
                                    sensitivity to storage time either before or after sampling,
                                    confirming that any fractionation due to permeation of noble
                                    gases across the double o-ring seals and through the
                                        N 2 filled necks and cavities was
                                    below analytical detection [6] . In the field, three well casing volumes were purged
                                    from each well prior to sampling. Flasks were first prepared for
                                    sampling by attaching 1.25-cm inner-diameter Tygon tubing to the
                                    outer neck of the flask and flushing the tubing up to the inner
                                    o-ring seal with N 2 gas flowing through
                                    0.3-cm Nylon tubing inserted into the Tygon tubing. With the
                                        N 2 gas flowing, 0.6-cm outer diameter
                                    Nylon tubing was connected to the groundwater pump and inserted
                                    into the Tygon tubing up to the inner o-ring seal. The 0.3-cm
                                    diameter tubing was then removed and the Tygon tubing was
                                    flushed with the groundwater, with care taken to dislodge any
                                    bubbles. At this point, sampling began by cracking open the
                                    Louwers-Hapert valve to allow groundwater to enter the evacuated
                                    flask while maintaining a buffer volume of groundwater in the
                                    neck and Tygon tubing to prevent any incorporation of
                                    atmospheric air. Once the flask was ~95% full, the
                                    Louwers-Hapert valve was closed and the cavity between the
                                    o-rings as well as the neck volume were filled again with
                                        N 2 gas and capped. Extraction and purification of dissolved gases At SIO, samples were weighed both before and after
                                    sampling for the purpose of determining bulk dissolved gas
                                    concentrations via manometry. Dissolved gases were
                                    quantitatively extracted from each sample by sparging with
                                    gaseous helium and cryogenically trapping liberated gases in a
                                    diptube immersed in a 4-K liquid helium
                                            dewar [6] . After a sample was
                                    initially connected via 0.5″ ultra-torr fittings to the
                                    extraction line, the space between the o-ring seal and vacuum
                                    line connection was evacuated to <0.1 mTorr and leak checked. Next, the sample was poured into a 6-L extraction vessel, which
                                    was initially under vacuum, and all remaining gases in the
                                    two-liter flask were cryogenically trapped over a 15-min period. At this point, the now-evacuated two-liter flask was closed off
                                    to the extraction line and 1 atm of ultra-high-purity helium gas
                                    was added to the entire line, connected to a flow-through
                                    diptube (in liquid helium) and recirculating Metal Bellows MB-41
                                    pump. Over a 90-min extraction period, the helium gas was
                                    recirculated at a 1 L min −1 flow rate
                                    and the diptube was progressively lowered into the dewar to
                                    prevent saturation of available surface area for gas trapping. After this period, helium gas was pumped away and the diptube
                                    was closed off and removed from the liquid helium dewar. Repeated testing of this extraction technique demonstrated that
                                    99.7 ± 0.1% of dissolved gases were
                                            extracted [6] . For each sample,
                                    extracted gases were gettered both by SAES Zr/Al sheets and Ti
                                    sponge for 130 min at 900 °C to remove all reactive gases. The
                                    remaining (noble) gases were then cryogenically transferred into
                                    another diptube immersed in liquid helium. Isotope-ratio mass spectrometry After allowing at least 3 h at room temperature for
                                    homogenization, the gases in the diptube were expanded into a
                                    calibrated volume attached to the inlet of a Thermo-Finnigan MAT
                                    253 isotope-ratio mass spectrometer and total pressure was
                                    measured using a 100-Torr Baratron capacitance manometer. With
                                    knowledge of the sample weight, total (noble) gas pressure,
                                    volume, and measurement temperature, dissolved Ar concentrations
                                    were calculated by making a slight correction in all samples for
                                    the presence of Ne (the most abundant of the other noble gases,
                                    representing ~0.1% of total noble gas pressure) and gas
                                    non-ideality using the second Virial
                                            coefficient [31] . The sample was then
                                    introduced to the bellows of the mass spectrometer and given
                                    10 min for homogenization before analysis. Over a ~9-h analysis
                                    period, isotope ratios of Ar, Kr, and then Xe were measured in
                                    sequence with multi-collector Faraday cups, followed by
                                    elemental ratios (Kr/Ar and Xe/Ar) via peak jumping. Dissolved
                                    isotope and elemental ratios were measured dynamically against a
                                    working standard gas [19] . 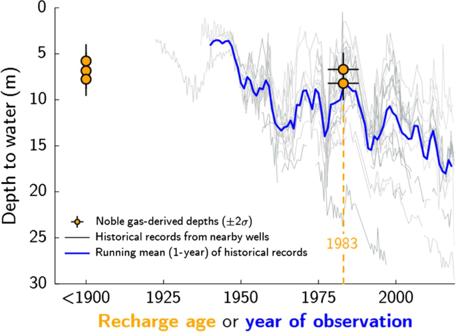Fig. 3: Modern validation of noble gas
                                                  isotope-derived water table depths. Water-table depth estimates derived from
                                                  groundwater noble gas isotope measurements are
                                                  compared to historical water-level observations
                                                  near two adjacent wells sampled in March 2018 near
                                                  Fresno, California. Depths are relative to the
                                                  land surface. Historical records from within a
                                                  10-km radius of the sample site were included,
                                                  except for those from the highly populated city
                                                  center, which dropped substantially in the
                                                  mid-20th century (Supplementary Fig.4). Multiple age
                                                  tracers were used to determine probable recharge
                                                  ages (Supplementary Fig.5). 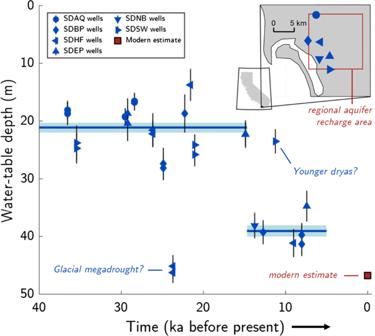Fig. 4: Reconstructed water-table depths in the San
                                                  Diego region. Noble gas isotope-derived water-table
                                                  depths (WTD) from the San Diego aquifer system are
                                                  presented in meters below the land surface. Blue
                                                  markers and error bars (±2σ) indicate WTD derived
                                                  from individual samples collected from wells at
                                                  multiple depths at six sites (indicated by marker
                                                  shapes). Pre and post 15-ka mean WTDs (lines with
                                                  ±2-SE shaded regions) exclude two extreme WTD
                                                  observations that could reflect a previously
                                                  documented glacial dry period and wet Younger
                                                  Dryas stadial. The present-day mean WTD over the
                                                  assumed recharge area (inset) was estimated by a
                                                  high-resolution, observation-constrained
                                                  groundwater model (red square marker). Groundwater
                                                  age uncertainties are roughly ±2 ka (Supplementary
                                                  Note4). Atmospheric air samples
                                    were collected and analyzed against this same working standard
                                    to normalize all measured isotope and elemental ratios to the
                                    well-mixed atmosphere. Detailed overviews of analytical
                                    corrections and uncertainty are provided in Supplementary
                                        Note 1 .